Vesicle-based artificial cells as chemical microreactors with spatially segregated reaction pathways In the discipline of bottom-up synthetic biology, vesicles define the boundaries of artificial cells and are increasingly being used as biochemical microreactors operating in physiological environments. As the field matures, there is a need to compartmentalize processes in different spatial localities within vesicles, and for these processes to interact with one another. Here we address this by designing and constructing multi-compartment vesicles within which an engineered multi-step enzymatic pathway is carried out. The individual steps are isolated in distinct compartments, and their products traverse into adjacent compartments with the aid of transmembrane protein pores, initiating subsequent steps. Thus, an engineered signalling cascade is recreated in an artificial cellular system. Importantly, by allowing different steps of a chemical pathway to be separated in space, this platform bridges the gap between table-top chemistry and chemistry that is performed within vesicles. Chemical reactions and biological processes performed in lipid vesicles are of great importance in the expanding field of bottom-up synthetic biology. There are two ultimate goals of this field: (i) the design of artificial cell-like systems using chemical building blocks and (ii) the assembly of smart, bio-inspired ‘machines’ employing various types of chemistries for purposes such as drug delivery and the production of biomolecules. Some of the most significant achievements concerning vesicle-based protocells include the incorporation of basic forms of replication [1] , communication [2] , transport [3] , biomolecule synthesis [4] , protein–protein interaction networks [5] and metabolism, amongst others [6] , [7] , [8] , [9] , [10] , [11] . There have also been significant advances in developing chemical and biological microreactors, either in vesicle or droplet form, that contain simple chemical reactions [12] , [13] , [14] , [15] . In all of these cases, the confined chemistries within the vesicles can be said to be ‘one-pot’ processes: there is only one confined space in which the reagents must be added beforehand. This restriction is an inherent feature of vesicles and limits the scope of processes, that can be performed within them. Herein, we show that by using vesicles with multiple compartments, one can define and control the spatial organization of content, allowing more elaborate multi-step reaction systems to be incorporated. Spatial segregation of content in compartments—and the subsequent interaction between these compartments—is key if the aforementioned goals of the field are to be achieved. Compartmentalization of content and function is a recurring characteristic in biology, most evidently in bacterial microcompartments and eukaryotic organelles [16] . Introducing such organizations into artificial cells will allow some universal features to be recreated. One such feature is a signalling cascade, a sequence of chemical reactions where each stage processes the output of the previous one. They are used by cells to sense their environment and to relay information between different cellular regions. In addition, segregation of content will allow regions to be optimized for specific purposes—for example, by the presence of reactants or specific chemical conditions—thus increasing the overall efficiency of the system. The analogy of a factory with different units performing distinct roles is applicable here. For these reasons, increasing attention has been paid to compartmentalized structures that host biochemical reactions. Most efforts have focussed on polymersomes [17] , [18] , [19] , which lack the biological relevance of lipids, and have a diminished ability for functionalization with biological components (protein pores, receptors, antibodies and so on). They also do not possess the rich phase behaviour that lipids do, which can be taken advantage for the introduction of responsiveness. Others have developed vesicles-in-vesicles, with the sequential release of inner-vesicle content, to achieve multi-step reactions [20] . However, the lack of defined spatial organization of content and the absence of connectivity between the inner vesicles is detrimental to their potential use and applications. Further, they do not employ membrane proteins for content release, relying instead on vesicle phase transitions. There have also been elegant methods to form networked vesicle nanoreactors, with nanotubes facilitating reagent transfer between regions [21] , [22] , [23] . However, these require manual manipulation of individual vesicles using expensive apparatus, and are therefore unsuitable for scale-up and for potential use as functional devices. Finally, the examples above lack the myriad advantages that droplet-based technologies offer, such as control over compartment size and content, high-throughput generation, potential for automation and so on [24] . Therefore, more suitable structures are required within which content can be confined in defined vesicle regions, to allow the spatial segregation of multi-step processes, and to enable communication between these regions. The recent development of the multi-compartment vesicle platform, a technique which we developed and characterized, addresses this need. These are vesicles that have partitioning lipid bilayers separating their internal volumes into several distinct compartments [25] . We construct such vesicles and have incorporated within them an engineered three-step chemical reaction pathway, each step mediated by a specific enzyme, and isolated in a distinct compartment. Communication between compartments is facilitated by the transmembrane protein pore alpha-hemolysin (α-HL), allowing the products of each step to traverse through the bilayer to initiate subsequent steps. In this way, chemical signals are propagated between defined vesicle regions, and an enzymatic cascade network is thus recreated in an artificial cell. Experimental system Multi-compartment vesicles were constructed by transferring a set number of water-in-oil droplets from an oil to an aqueous solution, a procedure known as phase transfer ( Fig. 1 ). This process—which is driven by the density difference between the droplets and the underlying oil and aqueous solutions—engulfs multiple droplets in a bilayer leading to vesicles with multiple compartments. The number and content of compartments were not stochastically determined, but were precisely defined beforehand with full user control. By only expelling a set number of droplets with predefined composition, the desired vesicle arrangement was reliably formed (for example, to generate a three-compartment vesicle, only three droplets were expelled). 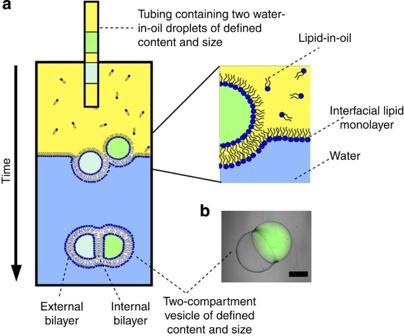Figure 1: Multi-compartment vesicle formation via the phase transfer of multiple droplets. (a) A set number of sucrose-loaded, lipid-coated water-in-oil droplets of defined composition are expelled above the same location of a water/oil column stabilized with a lipid monolayer. The droplets sink together through the column due to their higher density and deform the water–oil interface as they enter the aqueous phase. The interfacial monolayer envelops the lipid-coated droplets, encasing the droplets in a bilayer. (b) Brightfield/fluorescence composite of a two-compartment vesicle with predetermined compartment content. Scale bar, 250 μm. Figure 1: Multi-compartment vesicle formation via the phase transfer of multiple droplets. ( a ) A set number of sucrose-loaded, lipid-coated water-in-oil droplets of defined composition are expelled above the same location of a water/oil column stabilized with a lipid monolayer. The droplets sink together through the column due to their higher density and deform the water–oil interface as they enter the aqueous phase. The interfacial monolayer envelops the lipid-coated droplets, encasing the droplets in a bilayer. ( b ) Brightfield/fluorescence composite of a two-compartment vesicle with predetermined compartment content. Scale bar, 250 μm. Full size image The reaction system we employed had three distinct steps, each mediated by an enzyme ( Fig. 2a ). Step (1) is the transformation of lactose into glucose by lactase. Step (2) is the oxidation of glucose using glucose oxidase yielding H 2 O 2 . Step (3) is the oxidation of Amplex Red by H 2 O 2 in the presence of horseradish peroxidase (HRP), yielding a fluorescent molecule, resorufin. Each step of this multi-component pathway was isolated in a distinct compartment separated from one another by a lipid bilayer. 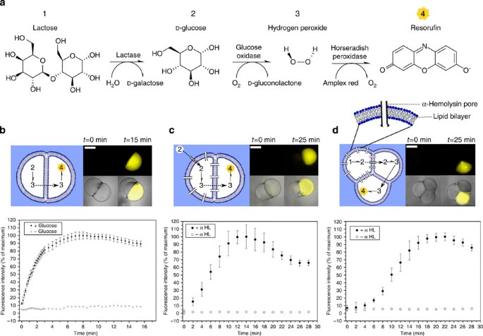Figure 2: Spatially segregated reaction sequences in multi-compartment vesicles. (a) Multi-step enzymatic pathway scheme (b-d) Schematic of the three vesicle systems that were generated, together with fluorescence and composite images of representative vesicles at the start and at the end of the reaction. Brightness and contrasts enhanced equally across all images. Scale bar, 250 μm. Graphs showing fluorescence intensity of the Amplex Red-containing compartment show the dye being oxidized to fluorescent resorufin as the reaction proceeds. (b) Glucose is oxidized, producing hydrogen peroxide, which translocates through the bilayer to initiate the oxidation of Amplex Red. (c) Glucose diffuses in from the exterior, through α-HL pores, to initiate subsequent reaction steps. This represents a simple sense/response network. (d) The full three-step reaction cascade where each step is isolated in a single compartment. Lactose is first hydrolysed to glucose, which then translocates through the bilayer to initiate subsequent steps as before. Error bars represent 1 s.d. (n=4). Figure 2: Spatially segregated reaction sequences in multi-compartment vesicles. ( a ) Multi-step enzymatic pathway scheme ( b - d ) Schematic of the three vesicle systems that were generated, together with fluorescence and composite images of representative vesicles at the start and at the end of the reaction. Brightness and contrasts enhanced equally across all images. Scale bar, 250 μm. Graphs showing fluorescence intensity of the Amplex Red-containing compartment show the dye being oxidized to fluorescent resorufin as the reaction proceeds. ( b ) Glucose is oxidized, producing hydrogen peroxide, which translocates through the bilayer to initiate the oxidation of Amplex Red. ( c ) Glucose diffuses in from the exterior, through α-HL pores, to initiate subsequent reaction steps. This represents a simple sense/response network. ( d ) The full three-step reaction cascade where each step is isolated in a single compartment. Lactose is first hydrolysed to glucose, which then translocates through the bilayer to initiate subsequent steps as before. Error bars represent 1 s.d. ( n =4). Full size image Spatially segregated enzymatic cascade We conducted a series of experiments showing the segregation of the various steps of the reaction pathway in multi-compartment vesicles. In each of these, we monitored the production of the reaction product resorufin (excitation 571 nm; emission 585 nm) using fluorescence microscopy. A schematic of the three experiments, together with graphs showing fluorescence increase over time and brightfield and fluorescence images of the vesicles is shown in Fig. 2 . In the first experiment, we encapsulated steps (2) and (3) of the reaction pathway in two-compartment vesicles ( Fig. 2b ). One compartment contained 0.25 M glucose and 2 U ml −1 glucose oxidase. The second contained 100 μM Amplex Red and 0.2 U ml −1 HRP. The product of the first step, H 2 O 2 , is permeable to lipid bilayers due to its small size (0.4 nm) and neutral charge [26] . For this reason, as soon as the vesicle was formed, an almost instantaneous fluorescence increase was seen in the second compartment: as H 2 O 2 diffused in, the second step was initiated and Amplex Red was oxidized yielding fluorescent resorufin. The reaction between H 2 O 2 , Amplex Red and HRP is rapid and the reaction went to completion within ~10 min [27] . In this case, H 2 O 2 can be thought of as a signalling molecule, mediating between the two steps (indeed, the role of H 2 O 2 as an intracellular signalling molecule is increasingly being recognized) [28] . The control experiment, where vesicles were identical apart from the absence of glucose, showed a constant and low fluorescence level, proving that H 2 O 2 was produced specifically by the action of glucose oxidase on glucose. In the next experiment, we wanted to show the initiation of the reaction cascade by an exogenous factor, namely the presence of 0.25 M glucose in the external solution ( Fig. 2c ). To do this, we generated two-compartment vesicles with glucose absent in the internal vesicle volume but present in the external solution. We also loaded the vesicles with 60 ng μl −1 α-HL monomers, which spontaneously insert into bilayers and aggregate to form heptameric protein pores (1.5 nm diameter) allowing glucose (molecular diameter of 1 nm) to diffuse through the pore [29] . This initiated the reaction, and a fluorescence increase was observed until a maximum intensity was reached after 22 min. It is noteworthy that the fluorescence increase was significantly slower than that of the previous experiment due to the requirement of glucose diffusion through the α-HL pores. The lack of fluorescence increase in the control scenario, where α-HL was not present, demonstrated that glucose originated from the external solution and was not present inside the vesicle. This example of an external stimulus instigating multi-step processes in different specialized compartments demonstrates the potential use of such systems for biosensing and therapeutic applications (for example, dormant systems being activated on encountering a biologically relevant stimulus for on-site drug synthesis). In the final experiment, we generated three-compartment vesicles and added a third step to the reaction. Steps (1), (2) and (3) were each isolated in distinct compartments ( Fig. 2d ). The first compartment contained 0.25 M lactose, 15 U ml −1 lactase and 60 ng μl −1 α-HL. The resulting hydrolysis product, glucose, passes through α-HL into the adjacent compartment containing glucose oxidase. As before, this initiated the next step in the cascade, with H 2 O 2 oxidizing Amplex Red to fluorescent resorufin in the third compartment. The fluorescence profile followed a similar pattern to the second experiment with the exception of a 6-min lag phase before fluorescence increase was observed. This is due to the time taken for the additional step, lactose hydrolysis by lactase, yielding glucose, to take effect. The control case, which was identical apart from the absence of lactose, showed no fluorescence increase over time, therefore demonstrating that glucose did indeed originate from lactose hydrolysis. In all the three experiments, a steady decrease in fluorescence was seen after peak fluorescence was reached. The principle reason for this is the leakage of fluorescent resorufin through the bilayers due to its partially hydrophobic character. Indeed, a fluorescence increase was seen in the adjacent compartments due to this leakage. This effect was compounded by a combination of photobleaching due to fluorescence exposure, and overoxidation of the product into non-fluorescent resazurin [27] . Vesicles were stable throughout the course of the experiments despite the high concentration of sucrose in their interiors. This was because immediately before droplet addition, a 2.5-M sucrose solution was injected into the bottom of the well. This acted as cushion to stop the vesicles contacting the glass substrate (due to density differences) and also crucially reduced the osmotic imbalance between the vesicle interior and exterior. This also contributed to the high yield of successful vesicle generation (~71%, n =17). One issue concerning this system is the lack of specificity regarding the direction of reagent diffusion. Without electrically driven flow, α-HL will let material diffuse in both directions. In addition, once H 2 O 2 is generated, it will permeate through all bilayers and not just into the intended compartment, resulting in a gradual loss of reagents and intermediate. However, as the enzymes were too large to move across the protein pore, the basic principle of the system was not compromised: each step still only took place within a designated compartment. The implications of this work broadly fall into two categories. First, it bridges the gap between table-top chemistry and chemistry that can be performed within the confines of a lipid vesicle. In traditional bench chemistry, discrete chemical steps of multi-step reaction pathways are segregated in time: the steps are performed sequentially, one after the other. Different reagents can be added or removed in each step, and the reaction conditions can also be altered. However, when employing chemistry in confined structures such as vesicles, this is more problematic: it is difficult to manually influence and manipulate these systems, especially if they are intended to perform functions in inaccessible environments (for instance, in vivo ). By segregating the reaction steps in space, this issue can be circumvented: each step can take place in a distinct compartment containing the necessary reagents to perform that particular step. It also creates a potential for more advanced systems, where individual steps take place in different conditions, as is seen in multi-step organic syntheses. The second implication is most apparent in the context of bottom-up synthetic biology. Each compartment can be said to host one step of a signalling cascade, transmitting a signal from one compartment to the next via a series of intermediaries. Indeed, as in cells, a chemical signal is received from the environment, transmitted across a cell membrane and then propagated to different regions via an internal signalling network to produce a response—in this case, synthesis of a fluorescent molecule. Signalling networks such as these are ubiquitous in biological systems, yet this work represents the first time it has been incorporated in a synthetic cell-like system. It also fulfills the same function as organelles in eukaryotic cells, where distinct membrane-bound regions are specialized to perform specific tasks. In the case described here, each compartment is optimized to perform each reaction by inclusion of the enzyme catalyst. This work is conceptually related to work undertaken on droplet interface bilayer networks by ourselves and other researchers (indeed, droplet interface bilayers are the structural precursors to multi-compartment vesicles) [30] , [31] , [32] , [33] , [34] . These networks are electrical, not chemical, in their nature: electrical signals are processed and manipulated to yield devices such as transistors, batteries and half-wave rectifiers [33] , [35] , [36] . Such research demonstrates the ability of compartmentalized systems to produce collective properties greater than the sum of their parts, eventually giving rise to complex biomimetic attributes [37] . In producing chemical networks existing in physiological environments in the form of vesicles, the power of such systems can be realized in the realms of synthetic biology and bioengineering to generate functional biodevices. Chemical reactions in spatially segregated vesicles open up several avenues for commercial applications, most notably for in situ drug manufacture, and as multi-component biodevices that offer a chemical response to environmental stimuli. Future work will likely involve the development of microfluidic technologies to reduce the vesicle size and enable high-throughput production (as have successfully been employed in droplet interface bilayer network and polymersome generation) [19] , [31] , [37] . These, together with engineering vesicle response to more biologically relevant stimuli (antibodies or metabolites, for instance), are the key areas that need to be addressed to realize the ambitious goals of the proposed systems. In conclusion, we have designed and constructed a series of multi-compartment vesicle systems, which enable discrete steps of chemical reaction pathways to be segregated in space. These factory-like ‘protocell’ units—composed of lipids, metabolic and membrane proteins and small molecule substrates—have different compartments specializing in performing distinct tasks. The output of one of these compartments is passed on to the next, either by passive diffusion through the bilayer walls, or through protein pore conduits. The vesicles are also shown to be able to process exogenous chemical signals. This work demonstrates the ability of this new class of enclosed structure, the multi-compartment vesicle, to increase the scope of the chemistry that can be performed in vesicles and creates potential for more complex vesicle-based chemical factories to be used in physiological environments. Multi-compartment vesicle formation All lipids were purchased from Avanti Polar Lipids and were used without further purification. Glucose oxidase, HRP and Amplex Red were purchased from Life Technologies. Lactase, α-HL and all other chemicals were purchased from Sigma Aldrich. Multi-compartment vesicles were generated using the phase transfer of two or three droplets across a water–oil interface as described elsewhere [25] . Briefly, a 10 mg ml −1 solution of 1,2-dioleoyl-sn-glycero-3-phosphocholine (DOPC) lipid in a 75:25 mixture of hexadecane and mineral oil was prepared by sonication for 10 min at 50 °C. This solution (0.5 ml) was then deposited above 0.5 ml of 50 mM sodium phosphate buffer, pH 7.4. This two-phase ‘column’ was left to stand for 2 h to allow a densely packed lipid monolayer to self-assemble at the interface. Aqueous droplets, loaded with the appropriate reaction components in buffer, and with 1.75 M sucrose, were then incubated for 5 min in an oil bath consisting of the same lipid-in-oil solution. Immediately before the addition of the droplets, 0.1 ml 2.5 M sucrose solution was injected into the bottom of the well. Two or three droplets (each 0.1 μl) were pipetted in the same locality of the upper oil phase to generate two- or three-compartment vesicles, respectively. The droplets (1.60 g ml −1 ) were denser than both the oil (0.78 g ml −1 ) and the external buffer solution (1.01 g ml −1 ), which drove them to descend through the column (under Archimedes’ principle), being encapsulated in a bilayer as they entered the aqueous phase. As multiple droplets descended together, they were consequently encapsulated together, and multi-compartment vesicles were generated. The content of the droplets becomes the content of the vesicle compartment, as the former is a precursor of the latter. Importantly, molecular biology grade sucrose and lactose (BioUltra) was used to reduce to possibility of glucose contamination. To increase the stability of the structures, the starting droplets were also loaded with 10 mg ml −1 1,2-diphytanoyl-sn-glycero-3-phosphocholine (DPhPC) 100-nm liposomes, formed by extruding 11 times through a polycarbonate membrane. Fluorescence microscopy All experiments were viewed with a Nikon Eclipse TE2000-E inverted microscope. Fluorescence experiments used an illuminating mercury arc lamp, and were imaged with a tetramethylrhodamine filter, at an exposure time of 10 ms. The lamp was turned off after each acquisition event to minimize photobleaching. Images were taken with a QICAM camera (QImaging) and were analysedw using ImageJ software. How to cite this article: Elani, Y. et al . Vesicle-based artificial cells as chemical microreactors with spatially segregated reaction pathways. Nat. Commun. 5:5305 doi: 10.1038/ncomms6305 (2014).